System-wide identification of wild-type SUMO-2 conjugation sites SUMOylation is a reversible post-translational modification (PTM) regulating all nuclear processes. Identification of SUMOylation sites by mass spectrometry (MS) has been hampered by bulky tryptic fragments, which thus far necessitated the use of mutated SUMO. Here we present a SUMO-specific protease-based methodology which circumvents this problem, dubbed Protease-Reliant Identification of SUMO Modification (PRISM). PRISM allows for detection of SUMOylated proteins as well as identification of specific sites of SUMOylation while using wild-type SUMO. The method is generic and could be widely applied to study lysine PTMs. We employ PRISM in combination with high-resolution MS to identify SUMOylation sites from HeLa cells under standard growth conditions and in response to heat shock. We identified 751 wild-type SUMOylation sites on endogenous proteins, including 200 dynamic SUMO sites in response to heat shock. Thus, we have developed a method capable of quantitatively studying wild-type mammalian SUMO at the site-specific and system-wide level. Small Ubiquitin-like Modifier (SUMO) is a post-translational modification (PTM) of lysine residues in proteins, and plays a pivotal part in the regulation of many cellular processes ranging from transcription to genome maintenance and cell cycle control to the DNA damage response [1] , [2] , [3] , [4] , [5] , [6] . Precursor SUMO is processed by SUMO-specific proteases to generate mature SUMO [7] , which is subsequently conjugated to target proteins through an enzymatic cascade involving the dimeric E1-activating enzyme SAE1/2, the E2 conjugation enzyme Ubc9 and several catalytic E3 enzymes [8] . SUMOylation is often found to target lysines within the canonical consensus motif [VIL]KxE in proteins [9] , [10] . SUMOylation of proteins is a reversible process, since SUMO-specific proteases can efficiently remove SUMO from its target proteins [7] . SUMO is essential for the viability of all eukaryotic life, with the exception of some species of yeast and fungi [8] . Ubc9 knockout mice perish at the early post-implantation stage due to chromosome condensation and segregation defects [11] . More recently, SUMO-2 was found to be indispensable for the embryonic development of mice, whereas SUMO-1 and SUMO-3 knockout mice were still viable [12] . In humans, three different SUMOs are expressed; SUMO-1, SUMO-2 and SUMO-3. Mature SUMO-2 and SUMO-3 are nearly identical [13] . SUMO-1 only shares 47% sequence homology with SUMO-2/3, although all SUMOs are conjugated to their targets by the same enzymatic machinery. SUMO-2/3 are the more abundant forms of the SUMOs [14] . SUMO-1 is predominantly conjugated to RanGAP1. SUMO-1 and SUMO-2/3 share a significant overlap in conjugation targets, but also retain differential conjugation specificity [15] , [16] . Like other ubiquitin-like (Ubl) modifiers, SUMO is able to form polymeric chains by modifying itself [17] , [18] , an event that is upregulated under stress conditions such as heat shock [19] . Furthermore, SUMO can interact non-covalently with other proteins through SUMO Interacting Motifs (SIMs) [8] , [20] , [21] . An important example of this interaction is the SUMO-targeted Ubiquitin Ligase RNF4, which recognizes poly-SUMOylated proteins through its SIMs, and subsequently ubiquitylates these targets [22] , [23] . Additional examples of SIM-mediated interactions include the interaction between SUMO-modified RanGAP1 and the nucleoporin RanBP2 (ref. 24 ), and the localization of the transcriptional corepressor Daxx to PML nuclear bodies [25] . There is great interest in SUMO originating from various fields such as chromatin remodelling and the DNA damage response. SUMOylation has also become increasingly implicated as a viable target in a clinical setting [8] , [26] , [27] , [28] , [29] . In a screen for Myc-synthetic lethal genes, SAE1 and SAE2 were identified, indicative of Myc-driven tumours being reliant on SUMOylation [27] . Furthermore, SUMOylation is widely involved in carcinogenesis [29] . Nevertheless, the system-wide knowledge of protein SUMOylation is limited to the global protein level. Over the last decade, specific sites of SUMO modification have mainly been studied at the single protein level using low-throughput methodology. While proteomic approaches have elucidated hundreds of putative target proteins [15] , [19] , [30] , [31] , they have failed to elucidate SUMO acceptor lysines. Only recently, two studies have revealed a significant amount of SUMOylation sites under standard growth conditions as well as in response to various treatments [32] , and under heat stress conditions [33] . Increasingly powerful proteomics technologies have facilitated proteome-wide studies of PTMs [34] , [35] , [36] , [37] . Various well-studied major PTMs include phosphorylation [38] , [39] , acetylation [40] , methylation [41] and ubiquitylation [42] , [43] , [44] , [45] , [46] , where tens of thousands of endogenous modification sites have been identified at the system-wide level. However, site-specific identification of endogenous SUMOylation sites significantly trails behind these other PTMs. Besides unfavourable SUMOylation stoichiometry of proteins, the highly dynamic nature of the SUMO modification and technical difficulties in purifying SUMO from complex samples due to robust and efficient activity of SUMO proteases—the main problem is the cumbersome remnant that is situated on the target peptides after tryptic digestion. In mammalian cells, for all SUMOs, the tryptic remnant exceeds 3 kDa in size, greatly hampering the ability for modified peptides to be resolved from highly complex samples by current tandem mass spectroscopy (MS/MS) approaches. The most successful approaches in identifying SUMO acceptor lysines to date, have been through use of a mutant SUMO bearing a point mutation. These SUMO-2 mutants contain either the Q87R mutation, which is homologous to the sole yeast SUMO Smt3, or the T90R or T90K mutations, which are homologous to ubiquitin. In addition, all internal lysines could be mutated to arginines to render the mutant SUMO immune to Lys-C. In turn, this allows for pre-digestion of the entire lysate and enrichment of SUMOylated peptides as compared with proteins, greatly diminishing the sample complexity. These approaches have initially allowed for the identification of ∼ 200 SUMOylated lysines [47] , [48] , [49] , and more recently 1,000 sites in response to heat shock [33] , and over 4,000 sites in response to various cellular stresses [32] . Regardless of the success of approaches employing mutant SUMO, there are some drawbacks. First, the substitution of all internal lysines to arginines prevents the mutant SUMO itself from being modified, effectively abrogating the ability to form polymeric chains. SUMOylation sites can be mapped while using just the Q87R, but this hampers enrichment of modified peptides, a key step in the purification process for all other major PTMs. Usage of the T90K mutant allows peptide-specific enrichment through use of the diglycine antibody, but this method may result in false-positive identification of ubiquitin sites, and is incompatible with enzymes that cleave arginines at any stage. Second, the usage of mutant SUMO necessitates the usage of exogenous SUMO, and thus is incompatible with the identification of lysines modified by endogenous SUMO, for example, from clinical samples or animal tissues. We have successfully developed the PRISM methodology which circumvents the cumbersome tryptic SUMO remnant. PRISM involves chemical blocking of all free lysines in a complex sample, followed by treatment with SUMO-specific proteases, and subsequent identification of the ‘freed’ lysines by high-resolution MS. We identified 751 wild-type SUMOylation sites on endogenous proteins, characterized site dynamics in response to heat shock and confirmed six novel SUMO target proteins identified by PRISM. Thus, we provide a key step towards system-wide identification of endogenous protein lysines modified by wild-type SUMO in mammalian systems. SUMO-specific proteases are functional in stringent buffers To overcome the cumbersome tryptic fragment left after digestion of wild-type SUMO, a methodology was devised that utilizes SUMO-specific proteases to remove the SUMO, and then employs the ‘freed’ lysine as either a direct identifier or as an intermediate for chemical labelling (that is, by biotin). The first step in the development of the protocol, was finding buffer conditions stringent enough to lyse cells without loss of SUMOylation due to endogenous proteases. Furthermore, the buffer had to be compatible with the following steps, including chemical labelling of all lysines, function of recombinant SUMO protease, and function of trypsin. Urea was found to be highly efficient, and lysing HeLa cells in 8 M urea in the presence of acetamide swiftly and irreversibly inactivated all endogenous SUMO proteases ( Fig. 1 ). 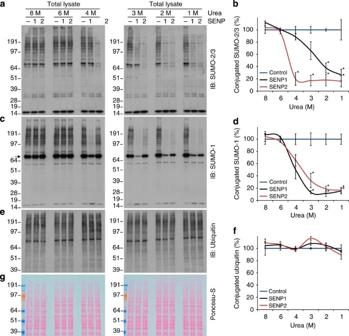Figure 1: SENP2 is able to cleave SUMO-2/3 from endogenous proteins in harsh buffer conditions. (a) HeLa cells were lysed in 8 M urea, homogenized and subsequently diluted to reduce the concentration of urea as indicated. Lysates were treated with SENP1, SENP2 or mock treated. After protease treatment, lysates were size-separated by SDS–PAGE, transferred to membranes, probed using a SUMO-2/3 antibody and visualized using chemiluminescence. The experiment was performed in biological triplicate. (b) As ina, and subsequently films were scanned and the amount of conjugated SUMO-2/3 was quantified and plotted against urea concentration.n=3, error bars represent s.e.m., asterisks indicate a significant difference as compared with control withP<0.01 by two-tailed Student’st-test. (c) As ina, but probed using a SUMO-1 antibody. SUMOylated RanGAP1 is indicated with an arrow. (d) As inb, but using a SUMO-1 antibody. (e) As ina, but probed using a ubiquitin antibody. (f) As inb, but using a ubiquitin antibody. (g) As ina, but with total protein content visualized using Ponceau-S staining. Figure 1: SENP2 is able to cleave SUMO-2/3 from endogenous proteins in harsh buffer conditions. ( a ) HeLa cells were lysed in 8 M urea, homogenized and subsequently diluted to reduce the concentration of urea as indicated. Lysates were treated with SENP1, SENP2 or mock treated. After protease treatment, lysates were size-separated by SDS–PAGE, transferred to membranes, probed using a SUMO-2/3 antibody and visualized using chemiluminescence. The experiment was performed in biological triplicate. ( b ) As in a , and subsequently films were scanned and the amount of conjugated SUMO-2/3 was quantified and plotted against urea concentration. n =3, error bars represent s.e.m., asterisks indicate a significant difference as compared with control with P <0.01 by two-tailed Student’s t -test. ( c ) As in a , but probed using a SUMO-1 antibody. SUMOylated RanGAP1 is indicated with an arrow. ( d ) As in b , but using a SUMO-1 antibody. ( e ) As in a , but probed using a ubiquitin antibody. ( f ) As in b , but using a ubiquitin antibody. ( g ) As in a , but with total protein content visualized using Ponceau-S staining. Full size image Subsequently, the HeLa lysate was diluted to lower concentrations of urea, and the activity of recombinant SENP1 and SENP2 was investigated. Strikingly, we found SENP2 to be able to cleave virtually all SUMO-2/3 from proteins at a concentration of 4 M urea ( Fig. 1a,b ). Under these conditions, SUMO-1 was not significantly affected by SENP2, and a further reduction to 3 M urea was required for SENP2 to efficiently cleave SUMO-1 off proteins ( Fig. 1c,d ). SENP1 was found to be less effective, only significantly affecting SUMO-2/3 at a concentration of 2 M urea, and SUMO-1 at a concentration of 3 M urea. SENP1 shows a slightly higher affinity for cleaving SUMO-1 as opposed to SUMO-2/3, but overall is less efficient than SENP2. Therefore, SENP2 was chosen as the main protease for identification of SUMO-2/3 sites. As controls, ubiquitin levels were investigated, and found to be completely unaffected by the SUMO proteases ( Fig. 1e,f ), and equal total protein levels were validated by Ponceau-S ( Fig. 1g ). To investigate the efficiency of SENP2 at removing SUMO-2/3 from proteins after heat shock, a similar assay was performed after HeLa cells had either been mock treated or subjected to heat shock. We observed no significant change in SENP2 activity towards SUMO-2/3, even though a large accumulation of SUMOylated proteins was observed in response to heat shock ( Fig. 2 ). As such, SENP2 can be efficiently employed to identify SUMO-2/3 sites in response to heat shock. 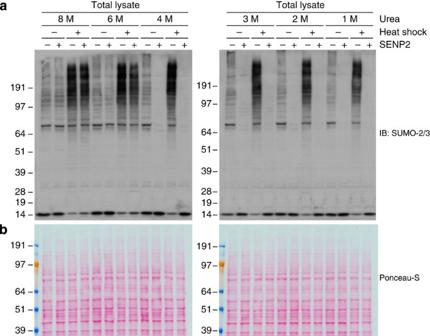Figure 2: SENP2 can process SUMOylation induced after heat shock under denaturing conditions. (a) HeLa cells were either incubated at 43 °C for 1 h or mock treated. Subsequently, the cells were lysed in 8 M urea, homogenized and subsequently diluted to reduce the concentration of urea as indicated.. Lysates were treated with SENP2 or mock treated. After protease treatment, lysates were size-separated by SDS–PAGE, transferred to membranes, probed using a SUMO-2/3 antibody and visualized using chemiluminescence. The experiment was performed in biological duplicate. (b) As ina, but with total protein content visualized using Ponceau-S staining. Figure 2: SENP2 can process SUMOylation induced after heat shock under denaturing conditions. ( a ) HeLa cells were either incubated at 43 °C for 1 h or mock treated. Subsequently, the cells were lysed in 8 M urea, homogenized and subsequently diluted to reduce the concentration of urea as indicated.. Lysates were treated with SENP2 or mock treated. After protease treatment, lysates were size-separated by SDS–PAGE, transferred to membranes, probed using a SUMO-2/3 antibody and visualized using chemiluminescence. The experiment was performed in biological duplicate. ( b ) As in a , but with total protein content visualized using Ponceau-S staining. Full size image SNHSA efficiently blocks all lysines in cellular lysates Following identification of a suitable SUMO protease, we endeavoured to find an efficient and affordable way of blocking all lysines in a complex sample. To this end, sulfosuccinimidyl-acetate (SNHSA) was used to block all lysines. SNHSA irreversibly acetylates all primary amines under alkaline buffer conditions, and is commercially available at relatively low cost. The efficacy of the compound was elucidated by treating HeLa total lysate with SNHSA, and subsequently digesting either mock-treated or SNHSA-treated lysate with endopeptidase Lys-C and trypsin. Samples were analysed by Coomassie to visualize total protein content, and SNHSA was observed to remarkably change the banding pattern of the HeLa lysate ( Fig. 3a ). Although many size shifts occurred, the banding pattern remained sharp after treatment with SNHSA, indicative of efficient and total labelling. Furthermore, digestion with endopeptidase Lys-C, which specifically cleaves C-terminal of free lysine residues, was found to be completely ineffective on SNHSA-treated HeLa lysate, demonstrating efficient protection of free lysines ( Fig. 3a ). Trypsin, which additionally cuts after arginines, was still able to fully digest both mock- and SNHSA-treated lysates. In addition, the effect of the SNHSA treatment on endogenous SUMO-2/3 was investigated. Similar to total protein levels, SNHSA-treated SUMOylated proteins were found to be resilient to digestion by Lys-C ( Fig. 3b ). Interestingly, we also observed an increase in SUMO signal after SNHSA treatment, which could be due to the SUMO-2/3 antibody more efficiently recognizing acetylated SUMO, or increased hydrophobicity of proteins altering immunoblotting behaviour. The ability of SENP2 to cleave fully acetylated SUMO-2/3 from completely acetylated proteins was confirmed ( Fig. 3c ). 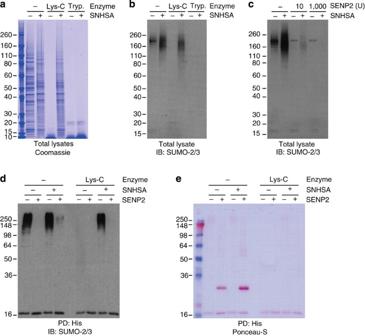Figure 3: SENP2 is able to remove acetylated SUMO from acetylated proteins after SNHSA treatment. (a) HeLa cells were lysed in 8 M urea, homogenized and subsequently treated with 10 mM SNHSA or mock treated. Next, both lysine-blocked and control samples were treated with either trypsin or Lys-C, or mock treated. All samples were size-separated by SDS–PAGE, and total protein content was visualized using Coomassie. The experiment was performed in biological duplicate. (b) As ina, but with samples transferred to membranes after SDS–PAGE, subsequently probed using a SUMO-2/3 antibody and visualized using chemiluminescence. (c) HeLa cells were lysed in 8 M urea, homogenized and subsequently treated with 10 mM SNHSA or mock treated. Next, both lysine-blocked and control samples were treated with either a standard or large amount of SENP2, or mock treated. All samples were size-separated by SDS–PAGE, transferred to membranes, probed using a SUMO-2/3 antibody and visualized using chemiluminescence. The experiment was performed in biological duplicate. (d) HeLa cells stably expressing lysine-deficient His10-tagged SUMO-2 were lysed and homogenized and subsequently SUMOylated proteins were enriched by Ni-NTA pulldown (PD:His). SUMOylated proteins were treated on-beads with SNHSA or mock treated, prior to elution. After elution, proteins were either treated with SENP2 or mock treated. Finally, samples were digested using Lys-C or mock digested. All samples were size-separated using SDS–PAGE, transferred to membranes, probed using a SUMO-2/3 antibody and visualized using chemiluminescence. The experiment was performed in biological duplicate. (e) As ind, but with total protein content visualized using Ponceau-S staining. Figure 3: SENP2 is able to remove acetylated SUMO from acetylated proteins after SNHSA treatment. ( a ) HeLa cells were lysed in 8 M urea, homogenized and subsequently treated with 10 mM SNHSA or mock treated. Next, both lysine-blocked and control samples were treated with either trypsin or Lys-C, or mock treated. All samples were size-separated by SDS–PAGE, and total protein content was visualized using Coomassie. The experiment was performed in biological duplicate. ( b ) As in a , but with samples transferred to membranes after SDS–PAGE, subsequently probed using a SUMO-2/3 antibody and visualized using chemiluminescence. ( c ) HeLa cells were lysed in 8 M urea, homogenized and subsequently treated with 10 mM SNHSA or mock treated. Next, both lysine-blocked and control samples were treated with either a standard or large amount of SENP2, or mock treated. All samples were size-separated by SDS–PAGE, transferred to membranes, probed using a SUMO-2/3 antibody and visualized using chemiluminescence. The experiment was performed in biological duplicate. ( d ) HeLa cells stably expressing lysine-deficient His10-tagged SUMO-2 were lysed and homogenized and subsequently SUMOylated proteins were enriched by Ni-NTA pulldown (PD:His). SUMOylated proteins were treated on-beads with SNHSA or mock treated, prior to elution. After elution, proteins were either treated with SENP2 or mock treated. Finally, samples were digested using Lys-C or mock digested. All samples were size-separated using SDS–PAGE, transferred to membranes, probed using a SUMO-2/3 antibody and visualized using chemiluminescence. The experiment was performed in biological duplicate. ( e ) As in d , but with total protein content visualized using Ponceau-S staining. Full size image Enrichment of SUMOylated proteins and lysine blocking To further optimize the protocol, the ability to apply the SNHSA labelling ‘on-beads’ was investigated during a pulldown. This allowed pre-enrichment of SUMOylated proteins prior to treatment, and furthermore allowed washing away of excess chemical after the blocking process, enabling subsequent steps. To this end, a cell line stably expressing His10-tagged SUMO-2 was utilized. Furthermore, for the purpose of unambiguous monitoring of SUMO levels during optimization of the protocol, lysine-deficient SUMO-2 was employed, which effectively abrogated internal SUMO acetylation and the resulting variability in immunoblot read-out. Pre-enrichment of His-SUMO by nickel-affinity chromatography could be efficiently combined with blocking of all lysines with SNHSA while on-beads ( Fig. 3d ). After treatment with SNHSA, acid elution was employed to prevent primary amines from being present in the elution fraction, and thus allowing for a second labelling step. More importantly, the effectiveness of recombinant SENP2 on enriched acetylated SUMOylated proteins was found to remain highly efficient ( Fig. 3d ). Ponceau-S staining additionally showed an efficient removal of SUMO from its target proteins, regardless of acetylation status and a resistance of acetylated SUMOylated proteins to Lys-C ( Fig. 3e ). Repurification of proteins deSUMOylated by SENP2 We investigated the possibility to benefit from the lysines ‘freed’ by SENP2 in two different ways, the first being by using the free lysine as a target for a second chemical treatment. Here sulfosuccinimidyl-SS-biotin (SNHSSSB) was employed, which functions in the same way as SNHSA. However, instead of an acetyl, SNHSSSB couples a biotin to the lysine, which is furthermore linked by a disulfide bridge. This then allowed for a second purification of proteins labelled by biotin, where they were previously modified by SUMO-2 ( Fig. 4a ). The efficacy of this approach was elucidated by monitoring total SUMO-2 throughout the procedure, as well as a known SUMO target protein, TRIM33. The initial step included enrichment of His10-SUMO-2, with acetylation performed on-beads. TRIM33 seemed to be less efficiently purified after acetylation ( Fig. 4b ), but total internal acetylation of the protein may have interfered with the antibody recognizing the protein. Coincidently, total SUMO levels were found to be similar regardless of acetylation, due to the use of lysine-deficient SUMO, and the SUMO antibody used for immunoblot recognizing an epitope that does not contain lysines ( Fig. 4c ). Following purification, both the control and acetylated samples were treated with SENP2. TRIM33 was efficiently deSUMOylated, regardless of acetylation state ( Fig. 4d ). Other SUMOylated proteins were also efficiently deSUMOylated ( Fig. 4e ). 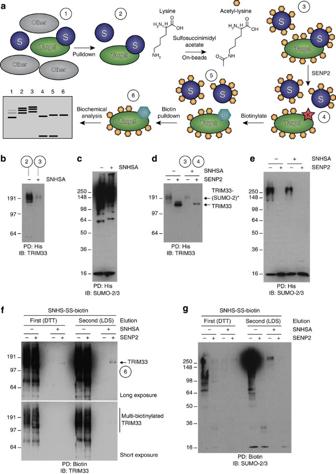Figure 4: A schematic overview of the PRISM double purification strategy. (a) 1. Cells are lysed under denaturing conditions, inactivating endogenous proteases. 2. SUMOylated proteins are pre-enriched using, in this case, Ni-NTA pulldown to capture the histidine tag. 3. SUMOylated proteins are acetylated on-beads using SNHSA under highly denaturing conditions, enabling efficient blocking of lysines. Proteins are eluted using a buffer compatible with a second chemical labelling step. 4. Following elution, lysine-blocked SUMOylated proteins are treated with SENP2, efficiently freeing up the lysines SUMO-2 was conjugated to. 5. Freed lysines are biotinylated using SNHSSSB. 6. Biotinylated SUMO target proteins are enriched using avidin pulldown, and eluted sequentially using DTT and LDS elution buffers. Finally, SUMO target proteins may be analysed by various biochemical methods, such as immunoblotting. (b) SUMOylated proteins were purified from HeLa cells expressing lysine-deficient His-tagged SUMO-2 (PD: His), using PRISM as described ina. For diagnostic reasons, the assay was performed with and without the use of SNHSA to block lysines. Samples were analysed by immunoblotting for the presence of TRIM33. Non-blocked TRIM33 eluted after Ni-NTA pulldown, Step 2, is indicated. Lysine-blocked TRIM33 eluted after Ni-NTA pulldown, Step 3, is indicated. The experiment was performed in biological duplicate. (c) As inb, but using a SUMO-2/3 antibody. (d) As inb, but additionally eluted proteins were either treated with SENP2 or mock treated. Lysine-blocked TRIM33 eluted after Ni-NTA pulldown, Step 3, is indicated. Lysine-blocked TRIM33 that was successfully deSUMOylated by SENP2, Step 4, is indicated. The experiment was performed in biological duplicate. (e) As ind, but using a SUMO-2/3 antibody. (f) All samples described indwere treated with SNHSSSB, and enriched using avidin pulldown (PD: Biotin). Elution was initially performed with DTT, and second with LDS. Samples were analysed by immunoblotting for the presence of TRIM33. On the long exposure, TRIM33 that was lysine-blocked, successfully deSUMOylated by SENP2 and specifically biotinylated and purified, Step 6, is indicated. On the short exposure, multi-biotinylated TRIM33 is indicated. The experiment was performed in biological duplicate. (g) Same as inf, but using a SUMO-2/3 antibody. Figure 4: A schematic overview of the PRISM double purification strategy. ( a ) 1. Cells are lysed under denaturing conditions, inactivating endogenous proteases. 2. SUMOylated proteins are pre-enriched using, in this case, Ni-NTA pulldown to capture the histidine tag. 3. SUMOylated proteins are acetylated on-beads using SNHSA under highly denaturing conditions, enabling efficient blocking of lysines. Proteins are eluted using a buffer compatible with a second chemical labelling step. 4. Following elution, lysine-blocked SUMOylated proteins are treated with SENP2, efficiently freeing up the lysines SUMO-2 was conjugated to. 5. Freed lysines are biotinylated using SNHSSSB. 6. Biotinylated SUMO target proteins are enriched using avidin pulldown, and eluted sequentially using DTT and LDS elution buffers. Finally, SUMO target proteins may be analysed by various biochemical methods, such as immunoblotting. ( b ) SUMOylated proteins were purified from HeLa cells expressing lysine-deficient His-tagged SUMO-2 (PD: His), using PRISM as described in a . For diagnostic reasons, the assay was performed with and without the use of SNHSA to block lysines. Samples were analysed by immunoblotting for the presence of TRIM33. Non-blocked TRIM33 eluted after Ni-NTA pulldown, Step 2, is indicated. Lysine-blocked TRIM33 eluted after Ni-NTA pulldown, Step 3, is indicated. The experiment was performed in biological duplicate. ( c ) As in b , but using a SUMO-2/3 antibody. ( d ) As in b , but additionally eluted proteins were either treated with SENP2 or mock treated. Lysine-blocked TRIM33 eluted after Ni-NTA pulldown, Step 3, is indicated. Lysine-blocked TRIM33 that was successfully deSUMOylated by SENP2, Step 4, is indicated. The experiment was performed in biological duplicate. ( e ) As in d , but using a SUMO-2/3 antibody. ( f ) All samples described in d were treated with SNHSSSB, and enriched using avidin pulldown (PD: Biotin). Elution was initially performed with DTT, and second with LDS. Samples were analysed by immunoblotting for the presence of TRIM33. On the long exposure, TRIM33 that was lysine-blocked, successfully deSUMOylated by SENP2 and specifically biotinylated and purified, Step 6, is indicated. On the short exposure, multi-biotinylated TRIM33 is indicated. The experiment was performed in biological duplicate. ( g ) Same as in f , but using a SUMO-2/3 antibody. Full size image Subsequently, all samples were treated with SNHSSSB, and an avidin pulldown was performed to enrich biotinylated proteins. The elution was performed in two steps, first with dithiothreitol (DTT) to specifically cleave the disulfide bridges and elute proteins without the biotin remnant, and second with LDS to achieve total elution. TRIM33 was used as a SUMO target to validate the methodology. After performing the entire assay in the intended manner, we confirmed TRIM33 by immunoblot as a single band ( Fig. 4f ). When skipping the initial acetylation step with SNHSA, we observed a large accumulation of multiply biotinylated TRIM33 proteins as a result of the large amount of free lysines in the protein. Due to use of a limited amount of SNHSSSB, the reaction could not complete full biotinylation of TRIM33, resulting in the visible ‘smear’ of TRIM33 proteins ( Fig. 4f ). As anticipated, for total SUMO-2/3, immunoblot signal was only observed when neither acetylating nor deSUMOylating ( Fig. 4g ). Overall, we demonstrated the ability to highly specifically purify SUMO target proteins by initially capturing them through the presence of their SUMO, and then re-capturing them through the absence of their SUMO when removed by SENP2. Identification of lysines modified by wild-type SUMO-2/3 To extend the PRISM strategy to mapping SUMO-2/3 sites, the methodology was slightly altered. It should be mentioned that wild-type SUMO-2 was employed for all proteomics experiments. To this end, a HeLa cell line stably expressing a low level of His10-SUMO-2-IRES–GFP was generated. Characterization of this cell line demonstrates expression of a modest level of His10-tagged but otherwise wild-type SUMO-2/3 ( Fig. 5a ), and correct localization of His10-SUMO-2 in the nucleus of the cells ( Fig. 5b ). 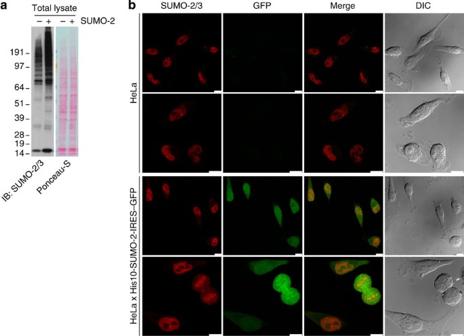Figure 5: Characterization of HeLa cells stably expressing a low level of His10-SUMO-2. (a) HeLa cells and HeLa cells stably expressing His10-SUMO-2 were harvested and lysed. Lysates were size-separated by SDS–PAGE, transferred to membranes, probed using a SUMO-2/3 antibody and visualized using chemiluminescence. Ponceau-S is shown as a loading control. The experiment was performed in biological duplicate. (b) HeLa cells and HeLa cells stably expressing His10-SUMO-2 were cultured on glass slides, fixed and immunostained for SUMO-2/3. Cells were investigated using confocal microscopy and immunostained SUMO-2/3 (red) and GFP (green) were visualized. Non-fused GFP is present due to expression of the His10-SUMO-2-IRES–GFP construct. The merged column is a combined display of SUMO-2/3 and GFP. Differential interference contrast (DIC, grey) scanning was performed to visualize the physical contours of the cells. Scale bars, 10 μm. Figure 5: Characterization of HeLa cells stably expressing a low level of His10-SUMO-2. ( a ) HeLa cells and HeLa cells stably expressing His10-SUMO-2 were harvested and lysed. Lysates were size-separated by SDS–PAGE, transferred to membranes, probed using a SUMO-2/3 antibody and visualized using chemiluminescence. Ponceau-S is shown as a loading control. The experiment was performed in biological duplicate. ( b ) HeLa cells and HeLa cells stably expressing His10-SUMO-2 were cultured on glass slides, fixed and immunostained for SUMO-2/3. Cells were investigated using confocal microscopy and immunostained SUMO-2/3 (red) and GFP (green) were visualized. Non-fused GFP is present due to expression of the His10-SUMO-2-IRES–GFP construct. The merged column is a combined display of SUMO-2/3 and GFP. Differential interference contrast (DIC, grey) scanning was performed to visualize the physical contours of the cells. Scale bars, 10 μm. Full size image PRISM was optimized for MS by leaving out the biotinylation and repurification step. Two concentration steps were also included to remove free SUMO from the samples ( Fig. 6a ). Stable Isotope Labelling of Cells (SILAC) was applied to ‘mark’ all proteins originating from the cell lysates and rule out contaminants. Both medium and heavy SILAC labelling was performed, and lysates were mixed in equimolar ratio immediately after cell lysis. In addition to a standard growth condition pool, a label-swapped experiment was performed where one of the two pools of cells (either medium or heavy) was heat shocked. After the initial enrichment and acetylation of SUMO-2 target proteins, the samples were concentrated over 100 kDa cut-off filters, specifically removing free unconjugated SUMO-2 ( Fig. 6b ). Subsequently, the samples were treated with SENP2 to cleave all SUMO-2 off the target proteins, followed by removal of SENP2 as well as SUMO-2, and another 100 kDa concentration step ( Fig. 6b ). It should be noted that concentration on 100 kDa filters under denaturing conditions of 8 M urea did not lead to any loss of proteins conjugated to SUMO-2, demonstrated here ( Fig. 6b ) and described previously [32] . 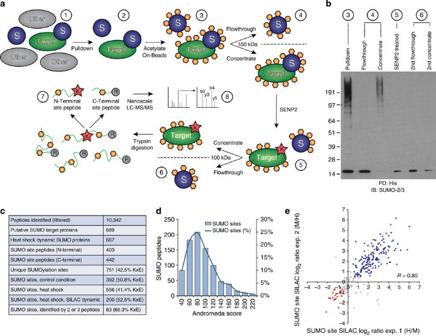Figure 6: PRISM combined with mass spectrometry reveals 751 unique SUMOylation sites. (a) A schematic overview of PRISM adapted to system-wide proteomics. 1. Cells are lysed under denaturing conditions, completely inactivating endogenous proteases. 2. SUMOylated proteins are pre-enriched using, in this case, Ni-NTA pulldown to capture the histidine tag. 3. SUMOylated proteins are acetylated on-beads using SNHSA under highly denaturing conditions, enabling efficient blocking of lysines. 4. Following elution, proteins are concentrated over a 100 kDa filter under denaturing conditions, specifically removing free SUMO but retaining SUMO-modified proteins. 5. Concentrated lysine-blocked SUMOylated proteins are treated with SENP2, efficiently removing SUMO-2 and freeing up the lysines SUMO-2 was conjugated to. 6. DeSUMOylated proteins are concentrated over a 100 kDa filter under denaturing conditions, removing SUMO cleaved off by SENP2 while retaining proteins that were previously SUMO modified. 7. Concentrated SUMO target proteins are trypsinized, with trypsin only able to cleave arginines and lysines that were freed by SENP2. Thus, two reporter peptides are generated per site, either ending in a lysine or preceded by a lysine. 8. Peptides are analysed using high-resolution mass spectrometry. (b) SUMOylated proteins were purified from medium and heavy SILAC-labelled HeLa cells stably expressing His-tagged SUMO-2 (PD: His), using PRISM as described ina. During various steps of the purification, samples were taken for diagnostic purposes. Samples were size-separated using SDS–PAGE, transferred to membranes, probed using a SUMO-2/3 antibody and visualized using chemiluminescence. Samples are indicated by the corresponding step number froma. The experiment was performed in SILAC label-swapped biological duplicate. (c) An overview of all identified peptides, putative SUMO target proteins, SUMO target proteins dynamic in response to heat shock and all reporter peptides mapping to unique SUMOylation sites. A small number of sites was identified by multiple reporter peptides. (d) A schematic overview of the Andromeda confidence scores for all peptides mapping to SUMOylation sites. (e) Scatter plot analysis depicting correlation between the SILAC log2ratios of all SUMO sites identified in the label-swapped heat shock experiment. Blue dots represent upregulated SUMO sites, and red dots represent downregulated SUMO sites. Pearson correlation is indicated. Figure 6: PRISM combined with mass spectrometry reveals 751 unique SUMOylation sites. ( a ) A schematic overview of PRISM adapted to system-wide proteomics. 1. Cells are lysed under denaturing conditions, completely inactivating endogenous proteases. 2. SUMOylated proteins are pre-enriched using, in this case, Ni-NTA pulldown to capture the histidine tag. 3. SUMOylated proteins are acetylated on-beads using SNHSA under highly denaturing conditions, enabling efficient blocking of lysines. 4. Following elution, proteins are concentrated over a 100 kDa filter under denaturing conditions, specifically removing free SUMO but retaining SUMO-modified proteins. 5. Concentrated lysine-blocked SUMOylated proteins are treated with SENP2, efficiently removing SUMO-2 and freeing up the lysines SUMO-2 was conjugated to. 6. DeSUMOylated proteins are concentrated over a 100 kDa filter under denaturing conditions, removing SUMO cleaved off by SENP2 while retaining proteins that were previously SUMO modified. 7. Concentrated SUMO target proteins are trypsinized, with trypsin only able to cleave arginines and lysines that were freed by SENP2. Thus, two reporter peptides are generated per site, either ending in a lysine or preceded by a lysine. 8. Peptides are analysed using high-resolution mass spectrometry. ( b ) SUMOylated proteins were purified from medium and heavy SILAC-labelled HeLa cells stably expressing His-tagged SUMO-2 (PD: His), using PRISM as described in a . During various steps of the purification, samples were taken for diagnostic purposes. Samples were size-separated using SDS–PAGE, transferred to membranes, probed using a SUMO-2/3 antibody and visualized using chemiluminescence. Samples are indicated by the corresponding step number from a . The experiment was performed in SILAC label-swapped biological duplicate. ( c ) An overview of all identified peptides, putative SUMO target proteins, SUMO target proteins dynamic in response to heat shock and all reporter peptides mapping to unique SUMOylation sites. A small number of sites was identified by multiple reporter peptides. ( d ) A schematic overview of the Andromeda confidence scores for all peptides mapping to SUMOylation sites. ( e ) Scatter plot analysis depicting correlation between the SILAC log 2 ratios of all SUMO sites identified in the label-swapped heat shock experiment. Blue dots represent upregulated SUMO sites, and red dots represent downregulated SUMO sites. Pearson correlation is indicated. Full size image Finally, the concentrated, acetylated and deSUMOylated proteins were digested with trypsin, and analysed using reversed-phase liquid chromatography (LC) followed by high-resolution MS. Since all lysines other than the ones freed by SENP2 are blocked, peptides ending in a lysine or peptides which would have been preceded by a lysine can be considered as SUMOylation sites. As an additional control, we performed a control experiment where we did not add SENP2 to the samples, and any peptides identified in this sample were considered as false positives. After initial filtering, we identified over 10,000 SILAC-labelled peptide pairs resulting from digested acetylated SUMO target proteins ( Fig. 6c and Supplementary Data 1 ). These peptides confidently map to nearly 700 putative SUMOylated proteins ( Supplementary Data 2 ), and we additionally found nearly 700 proteins to be dynamically SUMOylated in response to heat shock ( Supplementary Data 2 ), which is in line with numbers commonly found in the literature [15] , [19] , [31] , [49] . From all peptides, 8.2% contained a C-terminal lysine or were preceded by a peptide containing a C-terminal lysine. A similar number of both N-terminal (ending in a lysine) and C-terminal (preceded by a lysine) reporter peptides were found. Most of these reporter peptides had an Andromeda score in the range of 60–120 ( Fig. 6d ). After combining multiple peptides identifying the same site, we found 751 unique SUMOylation sites ( Supplementary Data 3 ), mapping to nearly 400 unique SUMOylated proteins ( Supplementary Data 4 ). The PRISM-identified SUMO sites displayed a 50.8% occurrence of the KxE consensus motif under standard growth conditions ( Fig. 6c and Supplementary Data 3 ), and a 41.4% KxE adherence in response to heat shock. When also considering KxD sites and the inverted SUMOylation motif [ED]xK, 63.1% of all sites matched consensus. About 83 SUMOylation sites were identified by 2 or 3 unique reporter peptides, providing a much higher identification confidence. We successfully quantified 274 SUMO sites by label-swapped SILAC, and found 200 of these sites to be dynamic in response to heat shock ( Fig. 6e ), with an overall very high Pearson correlation ( R =0.80). Properties of PRISM-identified SUMO sites and proteins The KxE frequency of sites identified with multiple reporter peptides was found to be 66.3%, because SUMOylation preferentially occurs on KxE sites, and increased stoichiometry of modification would facilitate more efficient purification and identification of multiple reporter peptides. To further ascertain the quality of the sites identified by PRISM, an IceLogo was generated, and the identified frequency of amino acids surrounding the SUMOylated lysines was compared with the randomly expected frequency ( Fig. 7a ). Here a strong enrichment for the SUMOylation motif [VIM]KxE was observed. Leucine at −1 was neither enriched nor depleted, and no enrichment of aspartic acid (D) at +2 was noted. Contrarily, enrichment of both glutamic and D was observed at −2, indicative of the inverted SUMO consensus motif [48] . Furthermore, enrichment of hydrophobic residues at −3 was found, indicative of the hydrophobic cluster motif [48] . A fill logo directly representing the frequency of all sequence windows was created, demonstrating the clear presence of the [VIL]KxE consensus ( Fig. 7b ). A heatmap corresponding to the IceLogo was generated, and displayed a clear enrichment of lysine and glutamic acid in the region surrounding the SUMOylation sites, indicative of solvent exposure ( Fig. 7c ). SUMO site sequence windows with an acid at −2 were compared with all other SUMO site sequence windows, and a significant depletion of the glutamic acid at +2 was observed ( Fig. 7d ). Thus, the inverted consensus motif is likely to function autonomously. 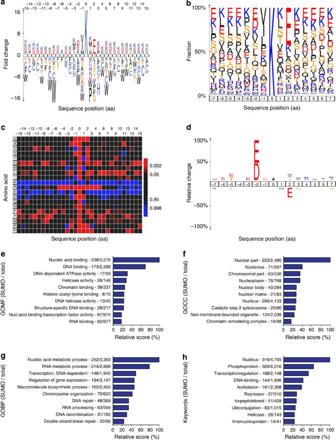Figure 7: Statistical analysis of SUMO sites and proteins. (a) IceLogo of all PRISM-identified SUMO-2 sites and their surrounding amino acids, ranging from −15 to +15 relative to the modified lysine. Amino acids indicated are contextually enriched or depleted as compared with randomly expected, with the height of the amino acids being representative of fold-change. All changes are significant withP<0.05 by two-tailed Student’st-test. (b) Fill Logo of all PRISM-identified SUMO-2 sites and their surrounding amino acids, ranging from −7 to +7, with the height of the amino acids directly correlating to percentage representation. (c) Heatmap representation ofa, giving a quick overview of enriched (blue) and depleted (red) amino acids surrounding SUMOylated lysines. Lysines and glutamic acids are enriched across the entire range surrounding SUMOylation. (d) Comparison of sequence windows of inverted SUMO sites (E or D at −2) to sequence windows of non-inverted SUMO sites. Amino acid height corresponds to percentage enrichment or depletion between the data sets representing inverted and non-inverted sites. Displayed amino acids are significantly different between the two data sets, withP<0.05 by two-tailed Student’st-test. (e) Term enrichment analysis, comparing all SUMO target proteins identified by PRISM to the human proteome. Gene Ontology Molecular Functions terms were used to find statistical enrichments within the SUMO target protein data set. Term enrichment score is a composite score based on enrichment over randomly expected and the negative logarithm of the false discovery rate. All listed terms are significant withP<0.02 by Fisher Exact testing. (f) As ine, using Gene Ontology Cellular Compartments. (g) As ine, using Gene Ontology Biological Processes. (h) As ine, using keywords. Figure 7: Statistical analysis of SUMO sites and proteins. ( a ) IceLogo of all PRISM-identified SUMO-2 sites and their surrounding amino acids, ranging from −15 to +15 relative to the modified lysine. Amino acids indicated are contextually enriched or depleted as compared with randomly expected, with the height of the amino acids being representative of fold-change. All changes are significant with P <0.05 by two-tailed Student’s t -test. ( b ) Fill Logo of all PRISM-identified SUMO-2 sites and their surrounding amino acids, ranging from −7 to +7, with the height of the amino acids directly correlating to percentage representation. ( c ) Heatmap representation of a , giving a quick overview of enriched (blue) and depleted (red) amino acids surrounding SUMOylated lysines. Lysines and glutamic acids are enriched across the entire range surrounding SUMOylation. ( d ) Comparison of sequence windows of inverted SUMO sites (E or D at −2) to sequence windows of non-inverted SUMO sites. Amino acid height corresponds to percentage enrichment or depletion between the data sets representing inverted and non-inverted sites. Displayed amino acids are significantly different between the two data sets, with P <0.05 by two-tailed Student’s t -test. ( e ) Term enrichment analysis, comparing all SUMO target proteins identified by PRISM to the human proteome. Gene Ontology Molecular Functions terms were used to find statistical enrichments within the SUMO target protein data set. Term enrichment score is a composite score based on enrichment over randomly expected and the negative logarithm of the false discovery rate. All listed terms are significant with P <0.02 by Fisher Exact testing. ( f ) As in e , using Gene Ontology Cellular Compartments. ( g ) As in e , using Gene Ontology Biological Processes. ( h ) As in e , using keywords. Full size image Finally, all PRISM-identified SUMO targets were matched to the annotated human proteome. Term enrichment analysis was performed to elucidate the overall functional characteristics and subcellular localization of this group of SUMOylated proteins ( Supplementary Data 5 ). For Gene Ontology (GO) Molecular Functions, the heaviest enrichment was found for nucleic acid, DNA- and RNA-binding categories ( Fig. 7e ). For GO Cellular Compartments, SUMOylated proteins were observed to be primarily located in the nuclear parts, and further enriched in the nucleoli, in the nuclear matrix, in nuclear bodies and at the chromatin ( Fig. 7f ). GO Biological Processes revealed involvement of SUMOylated proteins in nucleic acid metabolic processes, transcription regulation, DNA double-strand break processing and RNA splicing ( Fig. 7g ). Finally, a general keyword analysis revealed similar terms as the GO analyses, along with an enrichment of SUMOylation occurring on phosphorylated and acetylated proteins, as well as proteins involved in Ubl protein conjugation ( Fig. 7h ). A comparison of PRISM-identified SUMO sites and proteins To elucidate whether SUMOylated proteins as identified by PRISM are functionally related or interaction partners, an analysis using the Search Tool for the Retrieval of Interacting Genes/Proteins (STRING) database was performed [50] . Many of the identified SUMOylated proteins were situated in a single large STRING network ( Fig. 8a ). Overall, at a medium STRING confidence ( P >0.4), 86.0% of all identified proteins were tied together into a single cluster, with a ratio enrichment of 12.7 over randomly expected ( Fig. 8b ). At high STRING confidence ( P >0.7), 62.7% of all identified proteins still resided in the core cluster and the ratio enrichment over background increased further to 14.6. 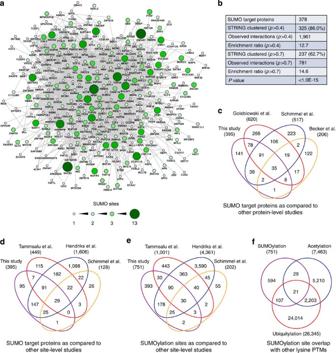Figure 8: A comparison of PRISM-identified SUMOylation sites and target proteins to other SUMOylation studies. (a) STRING network analysis of all PRISM-identified SUMO target proteins. The large majority of proteins formed one core cluster at STRING confidence of ≥0.4. The size and colour of the proteins is indicative of the amount of identified SUMOylation sites. (b) Statistical data supporting the STRING network analysis. STRING clustering was performed at STRING confidences of ≥0.4 and ≥0.7, separately. Enrichment ratio is the amount of observed interactions divided by the expected interactions, as provided by the online STRING database. (c) Four-way Venn diagram comparing PRISM-identified SUMOylated proteins to SUMO target proteins identified in three other studies. (d) Four-way Venn diagram comparing PRISM-identified SUMOylated proteins to SUMO target proteins identified in a site-specific manner in three other studies. (e) Four-way Venn diagram comparing PRISM-identified SUMOylated lysines to SUMOylation sites identified in three other studies. (f) Three-way Venn diagram comparing PRISM-identified SUMOylated lysines with all known ubiquitylation and acetylation sites. Figure 8: A comparison of PRISM-identified SUMOylation sites and target proteins to other SUMOylation studies. ( a ) STRING network analysis of all PRISM-identified SUMO target proteins. The large majority of proteins formed one core cluster at STRING confidence of ≥0.4. The size and colour of the proteins is indicative of the amount of identified SUMOylation sites. ( b ) Statistical data supporting the STRING network analysis. STRING clustering was performed at STRING confidences of ≥0.4 and ≥0.7, separately. Enrichment ratio is the amount of observed interactions divided by the expected interactions, as provided by the online STRING database. ( c ) Four-way Venn diagram comparing PRISM-identified SUMOylated proteins to SUMO target proteins identified in three other studies. ( d ) Four-way Venn diagram comparing PRISM-identified SUMOylated proteins to SUMO target proteins identified in a site-specific manner in three other studies. ( e ) Four-way Venn diagram comparing PRISM-identified SUMOylated lysines to SUMOylation sites identified in three other studies. ( f ) Three-way Venn diagram comparing PRISM-identified SUMOylated lysines with all known ubiquitylation and acetylation sites. Full size image Ambiguous identification of putative SUMOylated proteins may often lead to overestimation of a data set. As PRISM identifies proteins at the site level, interference from background proteins is greatly reduced. However, PRISM does not directly identify a site by modification on a peptide, and thus cannot benefit from the presence of reporter ions. Therefore, to further increase confidence of our data set, overlap analysis to other SUMOylation studies was performed. PRISM-identified proteins were compared with three major studies aimed at identification of SUMOylated proteins [15] , [19] , [49] , and 64.3% were found to be previously identified by these three studies ( Fig. 8c ). When also including putative SUMOylated proteins identified by Bruderer et al. [31] , this overlap further increased to 69.1% ( Supplementary Data 6 ). Comparatively, SUMO targets identified by Bruderer et al. [31] and Becker et al. [15] demonstrated significantly less overlap towards other studies. We found 21 SUMOylated proteins to be identified by PRISM and in all 4 aforementioned studies. When comparing PRISM to studies also identifying SUMOylated proteins by modification site [32] , [33] , [49] , 75.9% of all PRISM-identified SUMO targets previously had sites identified ( Fig. 8d and Supplementary Data 6 ). Next, PRISM-identified SUMO acceptor lysines were compared with SUMO sites previously mapped by these three other studies. Two of the studies utilized QQTGG mapping with either lysine-deficient Q87R SUMO-2 mutant under various growth conditions [32] , or otherwise wild-type Q87R SUMO-2 mutant at various stages of the cell cycle [49] . The third study used diglycine mapping with T90K SUMO-2 mutants under heat stress conditions [33] . A significant overlap between PRISM and the other three studies was observed, with 47.7% of all sites being previously identified in other screens ( Fig. 8e and Supplementary Data 7 ). Overlap was generally highly significant between all studies, with the smaller studies being increasingly enveloped by the larger studies. Finally, PRISM-identified SUMO sites were compared with known acetylation and ubiquitylation sites, and roughly one-fifth of the SUMOylation sites were found to be targeted by these other major lysine PTMs ( Fig. 8f ), indicating crosstalk. Finally, we observed modification of endogenous ubiquitin lysine-63 by wild-type SUMO-2 under standard growth conditions, and additionally lysine-6 and lysine-11 in response to heat shock, providing in vivo evidence for this novel hybrid Ubl chain. Confirmation of novel SUMO target proteins found by PRISM PRISM benefits from the unique property of generating peptides that differ greatly in size and sequence from standard trypsin-based approaches. As such, the technique can identify peptides and SUMO sites that are impossible to resolve using standard methods. After performing a comparison to other studies, we selected a subset of proteins, which were uniquely identified by PRISM at the SUMO site level, and performed pulldown and immunoblotting experiments to verify these SUMO targets. We enriched SUMO-2-modified proteins from both HeLa and U2OS cell lines expressing His10-SUMO-2. We investigated three proteins which were detected under standard growth conditions, PPIG, SSRP1 and TPR ( Fig. 9a ), and confirmed through immunoblotting that all three of these proteins were SUMO-modified in both HeLa and U2OS cells. Ponceau-S staining was performed to visualize input protein levels, and immunoblotting against SUMO-2/3 demonstrated efficient purification of SUMO-2 ( Fig. 9b ). 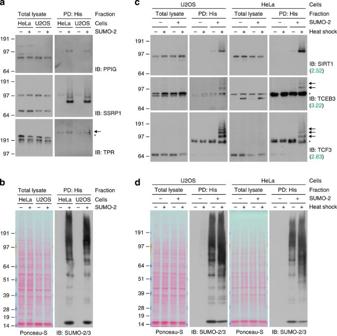Figure 9: Confirmation of PRISM-identified SUMO target proteins. (a) HeLa cells, HeLa cells stably expressing His10-SUMO-2, U2OS cells and U2OS cells stably expressing His10-SUMO-2 were harvested and lysed. SUMOylated proteins were purified using nickel-affinity chromatography. Total lysates and SUMO-enriched fractions (PD: His) were size-separated by SDS–PAGE, transferred to membranes, probed using the indicated antibodies and visualized using chemiluminescence. Asterisks indicate non-specific bands, and arrows indicate SUMOylated proteins. The experiment was performed in biological duplicate. (b) Controls fora, with Ponceau-S staining of total lysates as a loading control, and SUMO-2/3 immunoblot analysis of enriched fractions as a pulldown control. (c) As ina, with all cell lines incubated at 43 °C for 1 h or mock treated prior to lysis. SILAC heat shock response ratios (log2) are indicated. Asterisks indicate non-specific bands, and arrows indicate SUMOylated proteins. The experiment was performed in biological duplicate. (d) Controls forc, with Ponceau-S staining of total lysates as a loading control, and SUMO-2/3 immunoblot analysis of enriched fractions as a pulldown control. Figure 9: Confirmation of PRISM-identified SUMO target proteins. ( a ) HeLa cells, HeLa cells stably expressing His10-SUMO-2, U2OS cells and U2OS cells stably expressing His10-SUMO-2 were harvested and lysed. SUMOylated proteins were purified using nickel-affinity chromatography. Total lysates and SUMO-enriched fractions (PD: His) were size-separated by SDS–PAGE, transferred to membranes, probed using the indicated antibodies and visualized using chemiluminescence. Asterisks indicate non-specific bands, and arrows indicate SUMOylated proteins. The experiment was performed in biological duplicate. ( b ) Controls for a , with Ponceau-S staining of total lysates as a loading control, and SUMO-2/3 immunoblot analysis of enriched fractions as a pulldown control. ( c ) As in a , with all cell lines incubated at 43 °C for 1 h or mock treated prior to lysis. SILAC heat shock response ratios (log 2 ) are indicated. Asterisks indicate non-specific bands, and arrows indicate SUMOylated proteins. The experiment was performed in biological duplicate. ( d ) Controls for c , with Ponceau-S staining of total lysates as a loading control, and SUMO-2/3 immunoblot analysis of enriched fractions as a pulldown control. Full size image Similarly, we investigated three proteins we identified by modification site to be increasingly SUMOylated in response to heat shock. SIRT1, TCEB3 and TCF3 were all confirmed through immunoblot analysis to be increasingly SUMOylated in response to heat shock in HeLa and U2OS cells ( Fig. 9c ), demonstrating both reliable identification of SUMO sites and accurate quantification of heat shock dynamics using PRISM. Ponceau-S staining of input protein levels and immunoblotting against SUMO-2/3 were performed as controls ( Fig. 9d ). We have developed the PRISM methodology, which tackles the main problem that persisted in the MS field when trying to identify lysines modified by wild-type SUMO in mammalian systems. We demonstrated the efficacy of this novel methodology by successfully purifying known SUMO targets from a complex cell lysate. Furthermore, we combined PRISM with high-resolution MS, and identified 751 wild-type SUMOylation sites on endogenous protein lysines, purified from HeLa cells. About 35.5% adhered to the stringent [IVML]KxE consensus under standard growth conditions, and 63.1% were flanked by an acid residue at either −2 or +2. SUMOylated proteins were found to be predominantly nuclear, and involved in chromatin remodelling, RNA splicing, transcription and DNA repair. When compared with other SUMOylation studies, a significant overlap with PRISM-identified SUMO sites (48%) and SUMO target proteins (85%) was confirmed. We discovered one-fifth of the PRISM-identified SUMOylated lysines to overlap with ubiquitylation and acetylation. The observed modification of endogenous ubiquitin by wild-type SUMO-2 on lysine-63 suggests that SUMO-2 may be involved in blocking ubiquitin lysine-63 chain elongation. Our data set provides insight into the SUMO consensus motif and the functional groups of proteins being modified by SUMO, under standard growth conditions. Regardless, the data set is still fairly modest in size as compared with the other PTMs. The PRISM-identified sites were mapped to under 400 proteins, and using PRISM to identify sites across multiple cell types, and in response to multiple cellular treatments, will undoubtedly greatly increase global knowledge about SUMOylation. Compared with published studies on SUMO, PRISM not only provides the ability to identify wild-type SUMOylation sites, but also identified the third largest amount of total SUMO sites to date [32] , [33] , and the second largest amount of SUMO sites under standard growth conditions [32] . In total, 360 PRISM-identified sites were previously mapped by other studies. About 209 of these sites, or 58%, adhere to the KxE consensus. This is in most cases higher than the overall KxE identification rates for the studies separately, which range from 30 to 75% with the percentage becoming greater with a decreasing amount of total sites identified. Sites mapped by multiple approaches are far less likely to be false positives, and their repeated identification is in part a result from higher abundance in the purified samples. This is in agreement with the KxE motif being preferentially targeted by Ubc9 (refs 10 , 51 ), and SUMOylation on KxE motifs likely represents the lion’s share of total cellular SUMOylation under standard growth conditions. In response to heat shock, and by utilizing SILAC in a label-swapped experiment, we were able to quantify nearly 300 SUMOylation sites, and found 200 of these sites to be dynamically upregulated or downregulated in response to heat shock, with an above-average adherence to the KxE consensus motif of 53%. As such, PRISM can be used to quantitatively study wild-type SUMOylation at the site level. Overall, we observed multiple sites on the same proteins to be dynamically regulated in the same manner, although it should be noted that in response to heat shock the large majority of SUMO sites are upregulated. We investigated the efficacy of both SENP1 and SENP2 towards SUMO-1 and SUMO-2/3, and found SENP2 to be only significantly active towards SUMO-2/3 at a urea concentration of 4 M. As such, we utilized SENP2 for the identification of SUMO-2 sites in this manuscript, and we performed pre-enrichment of SUMO-2/3 prior to SUMO protease treatment. It should be noted that without such pre-enrichment, SENP2 could still feasibly be used as it does not efficiently target SUMO-1 under the correct buffer conditions. However, limited cross-reactivity cannot be excluded, which could yield false-positive identification of SUMO-1 sites as SUMO-2/3 sites, and as such extensive controls and pre-enrichment for the SUMO of interest are recommended. Similar approaches to PRISM, but then applied to different protein modifications, have been utilized in the last years. Notably, a study on acetylation was published that uses the biotin-switch methodology [52] , as well as a study on ubiquitin that uses the COFRADIC methodology [53] . While fundamentally similar, PRISM solves the tryptic remnant problem that has plagued the identification of endogenous SUMOylation sites. Contrarily, acetylation and ubiquitylation do not suffer from this limitation, and many thousands of acetylation and ubiquitylation sites have been published following a direct purification using an anti-acetyl-lysine antibody, or diglycine antibody, after tryptic digestion. While investigation of the specific activity of the protease in question remains of interest, the fidelity of these proteases in vitro is often not directly comparable to in vivo activity of these proteases. Furthermore, PRISM is performed under fully denaturing conditions, ensuring inactivation of all endogenous proteases, and allowing complete blocking of lysines in endogenous proteins. In addition, for identification of sites by MS, PRISM does not utilize biotinylation and subsequent purification, or any other method of relabelling the freed lysine. While this could be successful in reducing sample complexity, it does not address any potential background false-positive hits resulting from incomplete acetylation of lysines. To address this issue, we generated a false-positive control data set where the protease step was skipped. Here we found that the false-positive identification rate is just under 3%, with virtually all false-positive SUMO sites not matching the KxE consensus. Finally, leaving the lysine free after deSUMOylation allows for identification of two reporter peptides, due to trypsin being able to cleave the peptide, with both reporter peptides being shorter and thus easier to resolve. This is especially pivotal in the lysine-blocking context, already resulting in peptides that are on average twice as long as from a non-blocked tryptic digest. Interestingly, because SUMOylation sites are often situated in regions enriched for lysines ( Fig. 7a-c ), PRISM allows for identification of SUMOylated peptides that are lysine-rich up to the point where they would normally be unidentifiable due to being too short. Conclusively, PRISM can be utilized in a wider context to chart more wild-type SUMOylation sites in endogenous proteins, by investigation of different cell lines and in response to varying stimuli. The methodology is generic and is therefore widely applicable to study lysine PTMs. Ultimately, PRISM can be used to characterize wild-type SUMO sites in highly complex in vitro and in vivo samples. Plasmids The His10-SUMO-2 we described and used in this manuscript is based on Uniprot accession P55854 and has the following amino acid sequence: MAHHHHHHHHHHGGSM SEEKPKEGVKTENDHINLKVAGQDGSVVQF KIKRHTPLSKLMKAYCERQGLSMRQIRFRFDGQPINETDTPAQLEMEDEDTIDVFQQQTGG. His10-SUMO-2-K0-Q87R: MAHHHHHHHHHHGGSMSEERPREGVRTENDHINLRVAGQDGSVVQFRIRRHTPL SRLMRAYCERQGLSMRQIRFRFDGQPINETDTPAQL EMEDEDTIDVFRQQTGG. The corresponding nucleotide sequences were cloned in between the PstI and XhoI sites of the plasmid pLV-CMV-IRES–GFP [54] . Cell culture and cell-line generation HeLa cells were cultured in Dulbecco’s Modified Eagle’s Medium (DMEM) supplemented with 10% foetal bovine serum and 100 U ml −1 penicillin and streptomycin (Invitrogen). HeLa cell lines stably expressing wild-type His10-SUMO-2 and lysine-deficient His10-SUMO-2 (AllKR-Q87R mutant) were generated. To this end, HeLa cells were infected using a lentivirus encoding CMV-[SUMO]-IRES–GFP. Following infection, cells were sorted for low green fluorescent protein (GFP) fluorescence using a FACSAria II (BD Biosciences). All cell lines were tested for mycoplasma infection, and found to be clean. SILAC labelling for proteomic analysis For proteomics, HeLa cells stably expressing His10-SUMO-2 were seeded in 4 × 15-cm dishes containing either medium SILAC DMEM ([ 2 H 4 , 12 C 6 , 14 N 2 ]lysine/[ 13 C 6 , 14 N 4 ]arginine) or 4 × 15-cm dishes containing heavy SILAC DMEM ([ 13 C 6 , 15 N 2 ]lysine/[ 13 C 6 , 15 N 4 ]arginine), at a confluence of 25%. After 4 days of growth, all cells were trypsinized, washed twice with PBS and split to 10 × 15-cm dishes for both medium and heavy SILAC DMEM. Following an additional 4 days of growth, cells were either mock treated or incubated at 43 °C for 1 h. Subsequently, cells were harvested and lysed in 6 M guanidine-HCl, 100 mM sodium phosphate and 10 mM TRIS, pH 8.0. Lysates were sonicated at power 7.0 ( ∼ 30 W) for 2 × 5 s, using a microtip sonicator. Removal of SUMO using SUMO proteases in HeLa total lysate HeLa cells were harvested and lysed in 8 M urea and 100 mM sodium phosphate, pH 8.5. Chloroacetamide was added to 50 mM. Blocking of all lysines was performed by addition of SNHSA to a concentration of 20 mM, for 30 min at room temperature. Afterwards, TRIS pH 8.0 was added to a concentration of 50 mM. Urea dilutions were performed using 100 mM sodium phosphate, pH 8.5. Removal of SUMO was performed using recombinant catalytic domains of SENP1 and SENP2 (both purchased from LifeSensors). Digestion analysis of acetylated proteins was performed using Sequencing Grade Lys-C and Sequencing Grade Trypsin (both purchased from Promega). Enrichment of His10-SUMO-2 Lysates were supplemented with β-mercaptoethanol (β-ME) to a concentration of 5 mM, and imidazole (pH 8.0) to a concentration of 50 mM. About 20 μl Ni-NTA beads (Qiagen) were prepared per 1 ml of lysate, and subsequently washed (4 × ) and equilibrated in 6 M guanidine-HCl, 100 mM sodium phosphate, 10 mM TRIS, 5 mM β-ME and 50 mM imidazole, pH 8.0. Beads were added to lysates and tumbled for 5 h at room temperature. Beads were washed with the following buffers: Wash Buffer 1 (2 × ): 6 M guanidine-HCl, 100 mM sodium phosphate, 10 mM TRIS, 10 mM imidazole, 5 mM β-ME and 0.2% Triton X-100, pH 8.0; Wash Buffer 2 (4 × ): 8 M urea, 100 mM sodium phosphate, 5 mM β-ME and 0.2% Triton X-100, pH 8.0. On-beads lysine acetylation of His10-SUMO-2 proteins After the last wash with Wash Buffer 2, beads were resuspended in one bead volume of Acetylation Buffer (AB) supplemented by 20 mM SNHSA, and incubated for 10 min. AB is comprised of 8 M urea, 200 mM sodium phosphate, 5 mM β-ME, 0.2% Triton X-100 and 50 μg ml −1 phenol red (as pH read-out), pH 8.0. Next, a small amount of 6 M NaOH was added to raise the pH back up to 8. Following another 10 min incubation, a second bead volume of AB supplemented with 20 mM fresh SNHSA was added to the mixture. Samples were again incubated for 10 min, pH-adjusted to 8, and incubated for 10 min. Next, TRIS pH 8.0 was added to 20 mM. Beads were then washed with the following buffers. For proteomic samples, Triton X-100 was left out. Wash Buffer 3 (2 × ): 8 M urea, 100 mM sodium phosphate, 5 mM β-ME and 0.2% Triton X-100, pH 8.0. Wash Buffer 4 (2 × ): 8 M urea, 100 mM sodium phosphate and 0.1% Triton X-100, pH 6.3. Elution of acetylated His10-SUMO-2-conjugated proteins For biotinylation: following the final wash, proteins were eluted off the beads using one bead volume of 8 M urea, 56 mM citric acid and 44 mM sodium citrate, pH 4.4 (elution buffer). Beads were eluted twice for 15 min, and elutions were pooled, neutralized to pH 8.0 by addition of 6 M NaOH and cleared by passage through 0.45 μm filter columns (MilliPore). For proteomics: following the final wash, proteins were eluted off the beads using one bead volume of 8 M urea, 100 mM sodium phosphate, 10 mM TRIS and 500 mM imidazole, pH 7.0. Beads were eluted twice for 15 min, and elutions were pooled and cleared by passage through 0.45 μm filter columns. Concentration of acetylated His10-SUMO-2-conjugated proteins For proteomics, purified acetylated His10-SUMO-2 conjugated proteins were concentrated on a 100 kDa cut-off filter (Vivacon 500, Sartorius Stedim). Concentration was performed at 8,000 r.c.f. at a controlled temperature of 20 °C. Samples were concentrated to a volume equal to approximately one-fortieth to one-hundredth of the starting volume. Specific removal of His10-SUMO-2 from proteins by SENP2 Samples were gently diluted to 3 M urea by addition of 4 volumes of 1.75 M urea and 100 mM sodium phosphate, pH 8.5. After dilution, DTT was added to 2 mM. Subsequently, per 15-cm plate of cells used, 2.5 μg (250 U) of recombinant His10-SENP2 catalytic domain was added to the samples. Samples were gently mixed and left for 24 h at room temperature, in the dark and undisturbed. For proteomic analysis only, the concentration of urea was raised back up to 8 M. His10-SENP2 and free His10-SUMO-2 were removed by incubating the samples for 30 min with an amount of Ni-NTA beads equal to the amount used during the first purification in the presence of 50 mM imidazole, and subsequent clearing of the samples by centrifugation through 0.45 μm filter columns. The samples were then concentrated on a 100 kDa filter, as described previously. Labelling of SENP2-cleared lysines with sulfo-NHS-SS-biotin After removal of all SUMO-2 from the proteins, samples were treated with 1 mg (0.83 mM) of SNHSSSB. Following 2 h of incubation at room temperature, TRIS pH 8.0 was added to a final concentration of 50 mM, and samples were incubated for another 30 min at 30 °C to quench any remaining SNHSSSB. Subsequently, the concentration of urea was increased to 5 M. Enrichment of biotinylated proteins About 200 μl of Neutravidin beads (Thermo) were washed (4 × ) and equilibrated in 8 M urea, 100 mM sodium phosphate, 10 mM TRIS and 0.2% Triton X-100, pH 8.5 (Neutravidin Wash Buffer). The equilibrated neutravidin beads were added to the samples and tumbled for 3 h at room temperature. Following incubation, the beads were washed 6 × with Neutravidin Wash Buffer. Finally, beads were eluted for 10 min at 30 °C with one bead volume of Neutravidin Wash Buffer supplemented with 100 mM of DTT. A secondary elution was performed using one bead volume 1 × LDS Sample Buffer (NuPAGE) supplemented with 100 mM DTT, for 15 min at 50 °C. Electrophoresis and immunoblot analysis Protein samples were size-fractionated on Novex 4–12% Bis-Tris gradient gels using MOPS running buffer (Invitrogen), or on home-made 10% polyacrylamide gels using TRIS-Glycine buffer. Size-separated proteins were transferred to Hybond-C membranes (Amersham Biosciences) using a submarine system (Invitrogen). Gels were Coomassie stained according to manufacturer’s instructions (Invitrogen). Membranes were stained for total protein loading using 0.1% Ponceau-S in 5% acetic acid (Sigma). Membranes were blocked using PBS containing 0.1% Tween-20 (PBST) and 5% milk powder for 1 h. Subsequently, membranes were incubated with primary antibodies as indicated, in blocking solution. Incubation with primary antibody was performed overnight at 4 °C. Subsequently, membranes were washed three times with PBST and briefly blocked again with blocking solution. Next, membranes were incubated with secondary antibodies (donkey-anti-mouse-HRP or rabbit-anti-goat-HRP, Pierce) for 1 h, before washing three times with PBST and two times with PBS. Membranes were then treated with ECL2 (Pierce) as per manufacturer’s instructions, and chemiluminescence was captured using Biomax XAR film (Kodak). A compilation of all uncropped images corresponding to all scans of gels, membranes and films displayed throughout this manuscript is available as Supplementary Figure 1 . Microscopy Cells were seeded on glass coverslips in 24-well plates at ∼ 40,000 cells per well, and fixed after 24 h by incubation for 15 min in 3.7% paraformaldehyde in PHEM buffer (60 mM PIPES, 25 mM HEPES, 10 mM EGTA and 2 mM MgCl2 pH 6.9) at 37 °C. Cells were washed twice with PBS, and permeabilized with 0.1% Triton X-100 for 10 min, washed with PBST and blocked using TNB (100 mM TRIS pH 7.5, 150 mM NaCl and 0.5% Blocking Reagent (Roche)) for 30 min. Cells were incubated with Mouse α SUMO-2/3 antibody (ab81371, Abcam, 1:500) in TNB for 1 h. Cells were washed five times with PBST, and indicated with secondary antibody (Goat α Mouse Alexa 488 (Invitrogen), 1:500) in TNB for 1 h. Subsequently, cells were washed five times with PBST and dehydrated using alcohol, prior to embedding them in Citifluor (Agar Scientific) containing 400 ng per μl DAPI (Sigma) and sealing the slides with nail varnish. Images were recorded on a Leica SP5 confocal microscope system using 488 and 561 nm lasers for excitation and a × 63 lens for magnification, and were analysed with Leica confocal software. Primary antibodies Primary antibodies used in this study were Mouse α SUMO-2/3, Mouse α SUMO-1 (33–2400, Zymed, 1:1,000), Mouse α Ubiquitin (P4D1, sc-8017, Santa Cruz, 1:500), Rabbit α TRIM33 (A301-060A, Bethyl, 1:1,000), Rabbit α PPIG (3803S, Cell Signaling Technology, 1:1,000), Rabbit α TCEB3 (3685S, Cell Signaling Technology, 1:1,000, Rabbit α TCF3 (D15G11, 2883P, Cell Signaling Technology, 1:1,000), Rabbit α SIRT1 (D1D7, 9475P, Cell Signaling Technology, 1:1,000), Rabbit α SSRP1 (E1Y8D, 13421S, Cell Signaling Technology, 1:1,000) and Rabbit α TPR (A300-826A, Bethyl, 1:1,000). Indicated dilutions were those used for probing immunoblots. Validation of antibodies is provided on the manufacturers’ websites and in Antibodypedia. In-solution digestion and desalting of the peptides Acetylated deSUMOylated proteins in 8 M urea were supplemented with ammonium bicarbonate to 50 mM. Reduction and alkylation were performed with 1 mM DTT and 5 mM chloroacetamide, for 30 min, respectively. Samples were then diluted fourfold using 50 mM ammonium bicarbonate. Subsequently, 1 μg of Sequencing Grade Modified Trypsin (Promega) was added to the samples. Digestion with trypsin was performed overnight, at room temperature, still and in the dark. In-solution digested peptides were desalted essentially as described previously [55] . LC-MS/MS analysis Samples were analysed by means of nanoscale LC-MS/MS using an EASY-nLC system (Proxeon) connected to a Q-Exactive (Thermo) using Higher-Collisional Dissociation fragmentation. Samples were eluted off a reversed-phase C18 column packed in-house, using either a 2 h or a 4 h gradient ranging from 0.1% formic acid to 80% acetonitrile/0.1% formic acid, at a flow rate of 250 nl min −1 . The mass spectrometer was operated in data-dependent acquisition mode using a top 5 or top 10 method. The resolution of full MS acquisition was 70,000, with an AGC target of 3e6 and a maximum injection time of 20 ms. Scan range was 300 to 1,400 m/z or 300 to 1,750 m/z . For tandem MS/MS, the resolution was 17,500 with an AGC target of 1e5 and a maximum injection time of 60 ms, 100 ms or 120 ms. An isolation window of 2.2 m/z was used, with a fixed first mass of 100 m/z . Normalized collision energy was set at 25 or 30%. Singly charged objects and objects with a charge >6 were rejected, and peptide matching was preferred. A 30-s or 45-s dynamic exclusion was used. Data processing The MS proteomics data have been deposited to the ProteomeXchange Consortium [56] via the PRIDE partner repository with the data set identifier PXD001798. Analysis of the raw data was performed using MaxQuant version 1.5.1.0 (refs 57 , 58 ). MS/MS spectra were filtered and deisotoped, and the 24 most abundant fragments for each 100 m/z were retained. MS/MS spectra were filtered for a mass tolerance of 6 p.p.m. for precursor masses, and a mass tolerance of 20 p.p.m. was used for fragment ions. Peptide and protein identification was performed through matching the identified MS/MS spectra versus a target/decoy version of the complete human Uniprot database, in addition to a database of commonly observed MS contaminants. Up to five missed tryptic cleavages were allowed, to compensate for extensive internal acetylation within peptides due to the PRISM methodology. Cysteine carbamidomethylation was set as a fixed peptide modification. Peptide pairs were searched with a multiplicity of 2, allowing medium labelled and heavy labelled SILAC peptides, with a maximum of six labelled amino acids. Medium peptides were set to be labelled with Arginine-6 (monoisotopic mass of 6.020129) and Lysine-4-Acetyl (monoisotopic mass of 46.035672). Heavy peptides were set to be labelled with Arginine-10 (monoisotopic mass of 10.008269) and Lysine-8-Acetyl (monoisotopic mass of 50.024763). Protein N-terminal acetylation, methionine oxidation and peptide N-terminal carbamylation were set as variable peptide modifications. Moreover, to allow identification of peptides ending in a ‘free’ lysine, a ‘negative’ weight acetyl (monoisotopic mass of −42.010565) was set as a variable peptide C-terminal lysine modification. Up to seven peptide modifications were allowed. Peptides were accepted with a minimum length of six amino acids, a maximum size of 4.6 kDa and a maximum charge of 7. The processed data was filtered by posterior error probability to achieve a protein false discovery rate (FDR) of <1% and a peptide-spectrum match FDR of <1%. Peptides ending with a lysine or being preceded by a lysine were assumed to be corresponding to previously SUMOylated lysines. Peptides were additionally filtered to have an Andromeda score of at least 40, and detected as both a medium and a heavy labelled SILAC peptide. All peptides identified in the negative control (lacking SENP2) were disqualified. SUMO sites were considered to be quantified by SILAC if detected in both label-swapped experiments, and considered dynamic with SILAC log 2 ratios in both individual experiments <−0.5 or >+0.5. For the purpose of quantification, multiple peptides reporting the same SUMO sites were median-averaged. Proteins for comparative analysis ( Supplementary Data 4 ) were only those containing at least one SUMO site. The putative list of SUMO target proteins ( Supplementary Data 2 ) is based on all proteins detected after His10-SUMO-2 pulldown under standard growth conditions, and was filtered so proteins were identified by at least two peptides, one unique peptide, and adhered to an internal medium/heavy SILAC ratio in between 2/3 and 3/2. The list of SUMO target proteins dynamically regulated by heat shock ( Supplementary Data 2 ) is based on all proteins detected by at least two peptides, one unique peptide, and adhering to a label-swapped SILAC log 2 ratio averaging <−1 or >+1, with both individual experiments <−0.5 or >+0.5. IceLogo and heatmap generation For SUMOylation site analysis of all identified sites, IceLogo software version 1.2 (ref. 59 ) was used to overlay sequence windows to generate a consensus sequence, which was compensated against expected occurrence (IceLogo). Heatmaps were generated in a similar manner to IceLogos. All amino acids shown as enriched or depleted are significant with P <0.05. Term enrichment analysis Statistical enrichment analysis for protein and gene properties was performed using Perseus version 1.5.0.15 (ref. 60 ). The human proteome was annotated with GO terms [61] , including Biological Processes (GOBP), Molecular Functions (GOMF) and Cellular Compartments (GOCC). Additional annotation was performed with keywords, GSEA, Pfam, KEGG and CORUM terms. SUMOylated proteins were compared by annotation terms to the entire human proteome, using Fisher’s exact testing. Benjamini and Hochberg FDR was applied to P values to correct for multiple hypotheses testing, and final corrected P values were filtered to be <2%. Final scoring of terms was performed by multiplying the log 2 of the enrichment ratio by the negative log 10 of the FDR, which allowed ranking of terms by both their enrichment and confidence. STRING network analysis STRING network analysis was performed using the online STRING database [50] , using all SUMOylated proteins as input. Protein interaction enrichment was performed based on the amount of interactions in the networks, as compared with the randomly expected amount of interactions, with both variables directly derived from the STRING database output. Visualization of the interaction network was performed using Cytoscape version 3.0.2 (ref. 62 ). SUMO target protein overlap analysis For SUMO target protein analysis, all proteins identified in this work with at least one SUMO site were selected. For comparative analysis, SUMO-2 target proteins were selected from Becker et al. [15] , Golebiowski et al. [19] , Bruderer et al. [31] and Schimmel et al. [49] . SUMO-2 target proteins identified by site were selected from Matic et al. [48] , Schimmel et al. [49] , Tammsalu et al. [33] , and Hendriks et al. [32] . Where required, gene IDs were mapped to the corresponding Uniprot IDs. Perseus software was used to generate a complete gene list for all known human proteins, and all identified SUMO target proteins from our study as well as the above-mentioned studies were aligned based on matching Uniprot IDs. SUMOylation and PTM site overlap analysis For comparative analysis, all SUMOylation sites identified by Matic et al. [48] , Schimmel et al. [49] , Tammsalu et al. [33] and Hendriks et al. [32] , were assigned to matching Uniprot IDs and sequence windows were parsed. Furthermore, all MS/MS-identified ubiquitylation sites and acetylation sites were extracted from PhosphoSitePlus ( www.phosphosite.org ; ref. 63 ), and sequence windows were assigned. For each data set, duplicate sequence windows were removed. Perseus software was used to generate a matrix where all sequence windows from all PTMs were cross-referenced to each other. How to cite this article: Hendriks, I. A. et al. System-wide identification of wild-type SUMO-2 conjugation sites. Nat. Commun. 6:7289 doi: 10.1038/ncomms8289 (2015). Accession Codes: The mass spectrometry proteomics RAW data have been deposited to the ProteomeXchange Consortium [56] , via the PRIDE partner repository with the data set identifier PXD001798 .